ATP-induced electron transfer by redox-selective partner recognition Thermodynamically unfavourable electron transfers are enabled by coupling to an energy-supplying reaction. How the energy is transduced from the exergonic to the endergonic process is largely unknown. Here we provide the structural basis for an energy transduction process in the reductive activation of B 12 -dependent methyltransferases. The transfer of one electron from an activating enzyme to the cobalamin cofactor is energetically uphill and relies on coupling to an ATPase reaction. Our results demonstrate that the key to coupling is, besides the oxidation state-dependent complex formation, the conformational gating of the electron transfer. Complex formation induces a substitution of the ligand at the electron-accepting Co ion. Addition of ATP initiates electron transfer by provoking conformational changes that destabilize the complex. We show how remodelling of the electron-accepting Co 2+ promotes ATP-dependent electron transfer; an efficient strategy not seen in other electron-transferring ATPases. Electrons with strong reducing power enable chemically demanding processes in nature. Coupling the energetically unfavourable electron transfer to an exergonic process, such as an ATPase reaction, may energize the electrons. This kind of energy transduction is found for key players of the biological carbon and nitrogen cycles and drives the chemistry behind nitrogenases, radical-dependent β,α-dehydratases, the related benzoyl-CoA reductases and different corrinoid-dependent methyltransferases [1] , [2] , [3] , [4] . The corrinoid and [4Fe4S] cluster-containing protein (CoFeSP) acts in the late steps of the Wood–Ljungdahl pathway enabling microbes to assimilate CO 2 in anoxic habitats. CoFeSP accepts a methyl group from a methyl-tetrahydrofolate-bound methyltransferase (MeTr) and transfers it to acetyl-CoA synthase, for which it cycles between the CH 3 -Co(III)- and Co(I)-active states. The Co(I) state of CoFeSP is prone to oxidation generating the inactive Co(II) state [5] . Recently, we identified an ATP-dependent reductive activator of CoFeSP, termed RACo [4] . RACo regenerates the active Co(I) state by coupling ATP hydrolysis to an electron transfer from its [2Fe2S] cluster to the Co(II) ion of CoFeSP. RACo and inactive Co(II)–CoFeSP form a tight complex, whereas the two active states of CoFeSP, Co(I) and CH 3 -Co(III), do not interact with the activator [4] . RACo is homologous to other reductive activators of corrinoid enzymes [6] , which are members of the ASKHA-ATPase family [7] . Nitrogenase reductase, also called Fe protein [8] , the activator of atypical dehydratases [9] and reductive activators of corrinoid enzymes proteins are the three principal types of ATPases coupling ATP hydrolysis to an energetically uphill electron transfer. All three proteins consist of an ATPase module and a Fe/S-cluster module linked to the ATPase site. How the energy is transduced from the ATPase site to induce electron transfer from its Fe/S-cluster site in these proteins is scarcely understood. The crystal structure of the activation complex at 2.5 Å presented in this work provides insights into the reductive activation of CoFeSP by RACo. Complex formation does not have an impact on all redox-active groups bound to the two proteins but does influence the ATPase activity of RACo. We provide evidence that interprotein electron transfer is gated by large conformational changes and suggest a mechanistic model in which complex dissociation induced by ATP binding triggers electron transfer to reactivate CoFeSP. Overall structure of the RACo:CoFeSP complex The asymmetric unit of the crystal contains two homodimers of RACo, each flanked on both sides by one CoFeSP molecule ( Fig. 1 ), in agreement with the RACo:CoFeSP stoichiometry found in solution [4] . Complex formation induces large structural rearrangements in both the proteins. The two cofactor-carrying domains of the large subunit of CoFeSP (CfsA) undergo large rearrangements ( Fig. 1b ). The [4Fe4S] cluster-binding domain rotates by ~90° around a loop connecting it to the (β/α) 8 barrel domain whereby its [4Fe4S] cluster is shifted by 42 Å. The cobalamin-binding domain turns by ~45° abolishing interactions between the corrin ring and the small subunit CfsB ( Fig. 1b ) and binds now to the surface of RACo ( Fig. 1a ). The [2Fe2S] cluster domain of RACo is invisible in all four RACo monomers in the asymmetric unit. 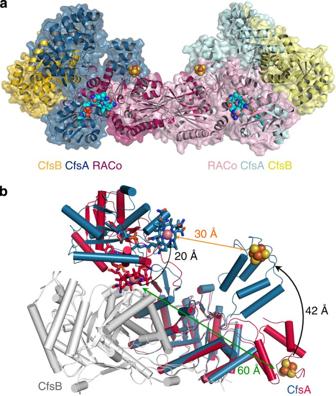Figure 1: Crystal structure of the RACo:CoFeSP complex. (a) Overall structure in cartoon and surface representation. The small (CfsB) and large (CfsA) subunit of CoFeSP are shown in yellow and blue, respectively. The RACo dimer is coloured in pink tones. The [4Fe4S] clusters of CoFeSP are illustrated as spheres in yellow (sulphur) and orange (iron). The cobalamin cofactor is depicted as cyan spheres. (b) Domain movements within CoFeSP. The structures of free CoFeSP (red, PDB2YCL)12and CoFeSP in the RACo:CoFeSP complex (blue) are superimposed on the small subunit CfsB (grey) to illustrate the domain movements in CfsA. A green (free CoFeSP) and an orange (complex) arrow indicate the distances between the [4Fe4S] cluster and the cobalamin cofactor. Black arrows point to the displacement of the cofactor-binding domains. Figure 1: Crystal structure of the RACo:CoFeSP complex. ( a ) Overall structure in cartoon and surface representation. The small (CfsB) and large (CfsA) subunit of CoFeSP are shown in yellow and blue, respectively. The RACo dimer is coloured in pink tones. The [4Fe4S] clusters of CoFeSP are illustrated as spheres in yellow (sulphur) and orange (iron). The cobalamin cofactor is depicted as cyan spheres. ( b ) Domain movements within CoFeSP. The structures of free CoFeSP (red, PDB 2YCL ) [12] and CoFeSP in the RACo:CoFeSP complex (blue) are superimposed on the small subunit CfsB (grey) to illustrate the domain movements in CfsA. A green (free CoFeSP) and an orange (complex) arrow indicate the distances between the [4Fe4S] cluster and the cobalamin cofactor. Black arrows point to the displacement of the cofactor-binding domains. Full size image We performed isothermal titration calorimetry experiments with Co(II)–CoFeSP, RACo and Δ100-RACo, a RACo variant devoid of the [2Fe2S] cluster domain ( Supplementary Fig. 1 ). From the nearly unchanged dissociation constants of the complex containing Δ100-RACo ( K D =6.7±0.8 nM) and full-length RACo ( K D =18.1±2.8 nM), we conclude that the [2Fe2S] cluster domain does not contribute to complex stabilization. Furthermore, resonance Raman spectroscopy did not reveal any change in the vibrational signature of the [2Fe2S] cluster [10] . Most likely, the [2Fe2S] cluster domain does not interact with other parts of the structure and is invisible in the crystal structure owing to its mobility. This flexibility of the [2Fe2S] cluster domain had already been observed in the structure of uncomplexed RACo [4] and seems to be retained in the RACo:CoFeSP complex. Cobalamin–RACo interaction Relocation of the cobalamin-binding domain towards RACo places the corrin ring in a newly formed pocket between the two ASKHA subdomains, where RACo surrounds the corrin ring on three of its four sides ( Fig. 2 ). The corrin ring fits tightly into the binding pocket, leaving no space for water molecules to approach the β-face of the corrin ring ( Fig. 2b ). The side chains of the corrin ring are engaged in a network of hydrogen bonds with the ASKHA domain ( Fig. 2a ). The numerous interactions between the corrin ring and RACo are in contrast to the few interactions between the corrin ring and the protein matrix found in the uncomplexed structure of CoFeSP. The water molecule acting as the β-ligand of Co(II) in free CoFeSP [11] , [12] is replaced by a serine residue from RACo (Ser398) ( Fig. 2a ). A stronger interaction of Co(II) with an axial ligand in the RACo:CoFeSP complex compared with free Co(II)–CoFeSP is in agreement with spectral changes observed upon complex formation by electron spin resonance (EPR) and resonance Raman spectroscopy [10] . 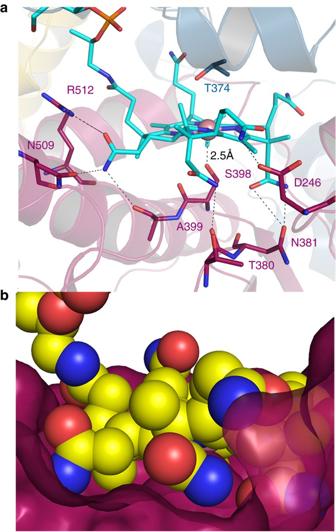Figure 2: Interactions of the cobalamin cofactor and RACo. (a) Residues of RACo (pink) interacting with the corrin ring (cyan stick model) are shown as sticks and interactions are denoted by black dashes. (b) Cobalamin (spheres) confined in the corrin-binding pocket of RACo (pink surface). Figure 2: Interactions of the cobalamin cofactor and RACo. ( a ) Residues of RACo (pink) interacting with the corrin ring (cyan stick model) are shown as sticks and interactions are denoted by black dashes. ( b ) Cobalamin (spheres) confined in the corrin-binding pocket of RACo (pink surface). Full size image The [4Fe4S] cluster domain is needed for complex formation The physiological role of the [4Fe4S] cluster of CoFeSP is enigmatic, as it does not directly contribute to the chemistry of methyl transfer neither from methyltransferase to CoFeSP nor from CoFeSP to acetyl-CoA synthase. It was suggested that the [4Fe4S] cluster was essential for the communication between CoFeSP and physiological electron donors providing a conduit for electron flow from, for example, CO-reduced carbon monoxide dehydrogenase or a ferredoxin to the cobalamin [13] , [14] . In the RACo:CoFeSP complex, the [4Fe4S] cluster domain of CoFeSP interacts extensively with the RACo dimer ( Supplementary Fig. 2a,b ). Accordingly, the RACo:CoFeSP complex is destabilized after deletion of the entire [4Fe4S] cluster domain (Δ60-CoFeSP) and was not detected by gel filtration chromatography ( Supplementary Fig. 3 ). Furthermore, electron transfer between Δ60-CoFeSP and RACo could not be initiated by the addition of ATP. Recently, a role of the [4Fe4S] cluster domain in complex formation was also described for the MeTr:CoFeSP complex structure of Moorella thermoacetica [15] . Although the structure and function of RACo and MeTr are completely different, CoFeSP interacts with both proteins using the same mobile domains to stabilize two different complexes ( Supplementary Fig. 4a ). In both cases, complex formation induces large movements of the two cofactor-carrying domains, displacing their bound metal sites by 6.5–14.8 Å in the MeTr:CoFeSP [15] and 20–42 Å in the RACo:CoFeSP complex ( Supplementary Fig. 4b ). Complex formation modulates the Co + reduction potential To gain insight on how the structural changes upon complex formation are reflected in the electron affinities of the cofactors, we performed a redox titration in combination with EPR spectroscopy and determined their redox potentials. While complex formation does not result in detectable changes of the redox potential of the [2Fe2S] cluster of RACo (−337 mV) and the [4Fe4S] cluster of CoFeSP (−560 mV), the midpoint potential of the Co(II)/Co(I) couple in free CoFeSP (−450 mV) shifts to a potential below −600 mV (most negative potential applied) in the complex ( Supplementary Fig. 5 ). This corresponds to a strong stabilization of the Co(II) state in the complex and is likely owing to the preference of each Co oxidation state for a different coordination number and geometry in cobalt complexes. While Co(I) favors a square-planar coordination by the corrin nitrogen atoms, additional axial ligands are found in the typically penta-coordinated Co(II) and hexa-coordinated Co(III) [16] . Thus, the interaction of the Co(II) ion with Ser398 ( Fig. 2a ) stabilizes the +II oxidation state explaining the lower electron affinity of Co(II) in the RACo:CoFeSP complex ( Supplementary Fig. 5 ). A stabilization of the inactive Co(II) state, however, seems to be contradictory to the function of RACo. Hence it appears mandatory for the reduction of Co(II) that the stabilizing β-ligand Ser398 dissociates to create the fourfold coordination favored in the Co(I) state. The open conformation of RACo In contrast to free RACo, which was observed in a closed conformation with a phosphate ion bound in a narrow cleft between the two ASKHA subdomains [4] , the ATP-binding site is wide open in the RACo:CoFeSP complex ( Fig. 3a,b ). Complex formation displaces the ASKHA subdomain II ( Fig. 3a ). This opening movement translates residues of subdomain II by up to 16 Å and results in the formation of various hydrogen bonds and salt bridges between subdomain II, CfsB and the cobalamin-binding domain of CfsA ( Supplementary Fig. 2c ). These interactions are not feasible in the closed conformation of RACo. The opening movement is also transmitted to the corrin-binding pocket of RACo, which is too narrow to fit the corrin ring in the closed conformation and opens upon complex formation ( Supplementary Fig. 6 ). Closed and open conformations have also been found for other members of the ASKHA family such as hexokinase [17] , the activator of 2-hydroxyacyl-CoA dehydratases [18] and Arp2/3 (ref. 19) [19] , where binding of Mg 2+ -ATP/ADP to the open conformation induces the closure of the ASKHA domain. Formation of the RACo:CoFeSP complex opens the ATP-binding site and stimulates the ATPase activity of RACo. While RACo alone has a specific activity of 1.58±0.19 mU (mg RACo ) −1 , the activity increases more than 20-fold to 38.12±5.44 mU (mg RACo ) −1 in the activation complex ( Supplementary Fig. 7 ). The higher ATPase activity reported for RACo previously [4] had masked this effect and was most likely owing to contaminating ATPases, which could be removed by a modified purification strategy including affinity chromatography for this study. 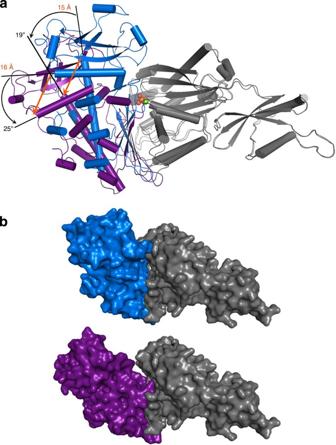Figure 3: Open and closed conformations of the ASKHA domain of RACo. (a) Superimposition of the closed (PDB3ZYY)4and open conformation of RACo. Only subdomain II of the ASKHA domain (residues 207–630) is presented in colour: free RACo in blue and CoFeSP-bound RACo in purple, respectively. Mg2+and PO43−bound to free RACo are shown as spheres. Orange arrows highlight the displacement of two helices. (b) Surface visualization of the open and closed conformation of RACo, coloured as ina. Figure 3: Open and closed conformations of the ASKHA domain of RACo. ( a ) Superimposition of the closed (PDB 3ZYY ) [4] and open conformation of RACo. Only subdomain II of the ASKHA domain (residues 207–630) is presented in colour: free RACo in blue and CoFeSP-bound RACo in purple, respectively. Mg 2+ and PO 4 3− bound to free RACo are shown as spheres. Orange arrows highlight the displacement of two helices. ( b ) Surface visualization of the open and closed conformation of RACo, coloured as in a . Full size image The following mechanism for the ATP-induced electron transfer between RACo and CoFeSP emerges from our results ( Fig. 4 ): in its free state, RACo has a closed ATP-binding site with a low basal ATPase activity, avoiding uncoupled ATP hydrolysis. CoFeSP protects its corrin ring and Co(II) by weak interactions between the cobalamin-binding domain and CfsB. Complex formation induces two large coupled conformational changes in RACo and CoFeSP ( Fig. 4 , i and ii). The movement of ASKHA subdomain II of RACo opens the ATP-binding site and the corrin-binding pocket ( Fig. 4 , ii). Opening of the ATP-binding site facilitates ATP binding and is responsible for the more than 20-fold ATPase activation observed in the activation complex. The open corrin-binding pocket allows a new conformation for the cobalamin-binding domain of CoFeSP and confines it by engaging the corrin ring in several interactions with RACo ( Fig. 4 , iii). Ser398 coordinates the Co(II) ion in the complex and stabilizes the Co(II) oxidation state. The redox-selective complex formation between RACo and CoFeSP [4] is explained by the potential of Co(II) in CoFeSP to accept Ser398 of RACo as β-ligand. In the active CH 3 -Co(III) state, the methyl group occupies the β-position, whereas the coordination site is non-bonding in the active Co(I) state. ATP addition triggers electron transfer [4] . As the RACo:CoFeSP complex is very stable (Δ G binding =−44 kJ mol −1 at 25 °C) ATP binding is needed to close the ASKHA subdomains and the corrin-binding pocket, which disrupts the interaction between RACo and CoFeSP and in turn splits the bond between Ser398 and Co(II) ( Fig. 4 , iv). Water molecules that could compensate for the lost coordination of Co(II) are excluded by the tight fit between the corrin ring and its binding pocket, forcing Co(II) to transiently adopt a square-planar Co(I)-like coordination, thus facilitating its reduction. Once Co(II) is destabilized, the reduced [2Fe2S] cluster of RACo provides its electron to produce active Co(I)–CoFeSP and oxidized RACo ( Fig. 4, v ). 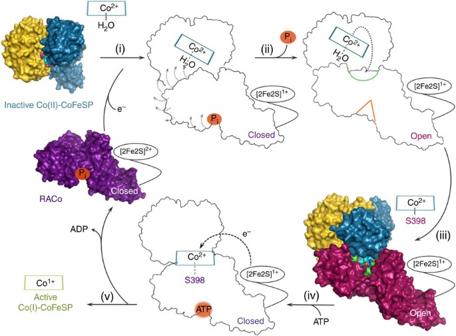Figure 4: Proposed mechanism of the ATP-induced reactivation of CoFeSP by its activator. Proteins are shown as surfaces. Intermediary states not captured in crystal structures are presented as contour plots, where the open ATP-binding site and corrin-binding pocket are indicated in green and orange, respectively and movements by dashed arrows. The corrin-binding pocket in the complex structure is shown in green. Complex formation between inactive Co(II)–CoFeSP and RACo in its closed conformation induces conformational changes in both proteins (i–iii). The ATP-binding site of RACo opens and the corrin-binding pocket is formed (ii). CoFeSP is now able relocate the cobalamin-binding domain and places the corrin ring into this pocket (iii). Ser398 replaces the water molecule as axial ligand and coordinates the Co ion in the activation complex (iii). For the stable complex to dissociate energy input is required. The binding of ATP causes the closure of the ASKHA subdomains and of the corrin-binding pocket disrupting the interaction between RACo and CoFeSP, especially between Ser398 and Co(II) (iv). In this transition state, the Co(II)-cobalamin adopts a square-planar Co(I)-like coordination facilitating the electron transfer from the reduced [2Fe2S] cluster of RACo to the accepting site resulting in reduced/active Co(I)–CoFeSP and oxidized RACo (v). Figure 4: Proposed mechanism of the ATP-induced reactivation of CoFeSP by its activator. Proteins are shown as surfaces. Intermediary states not captured in crystal structures are presented as contour plots, where the open ATP-binding site and corrin-binding pocket are indicated in green and orange, respectively and movements by dashed arrows. The corrin-binding pocket in the complex structure is shown in green. Complex formation between inactive Co(II)–CoFeSP and RACo in its closed conformation induces conformational changes in both proteins (i–iii). The ATP-binding site of RACo opens and the corrin-binding pocket is formed (ii). CoFeSP is now able relocate the cobalamin-binding domain and places the corrin ring into this pocket (iii). Ser398 replaces the water molecule as axial ligand and coordinates the Co ion in the activation complex (iii). For the stable complex to dissociate energy input is required. The binding of ATP causes the closure of the ASKHA subdomains and of the corrin-binding pocket disrupting the interaction between RACo and CoFeSP, especially between Ser398 and Co(II) (iv). In this transition state, the Co(II)-cobalamin adopts a square-planar Co(I)-like coordination facilitating the electron transfer from the reduced [2Fe2S] cluster of RACo to the accepting site resulting in reduced/active Co(I)–CoFeSP and oxidized RACo (v). Full size image How different energetic processes can be coupled is one of the recurring questions in bioenergetics and eminent in coupled electron transfers [20] . ATP-dependent electron transfer has been most extensively investigated for the two nitrogenase components [21] , [22] . Crystal structures of the nitrogenase complex with different nucleotides bound revealed large conformational changes on the electron-donating Fe-protein [23] , [24] . The electron-accepting metal clusters of the MoFe-protein are unperturbed in the known structures, but yet unobserved conformational changes on the MoFe-protein, which could gate electron transfer, appear plausible [25] . The energetic coupling strategy of RACo shows that manipulating the electron-accepting cofactor is a feasible way to gate an ATP-coupled electron transfer. This strategy is possible because RACo is able to access the metal ion in the electron-accepting cobalamin cofactor. The electron-accepting cofactors in nitrogenase and 2-hydroxyl-CoA dehydratase are FeS clusters, which are buried in the interior of the protein and cannot be accessed by the electron-donating ATPases. Therefore, different strategies are required in these systems. Our work on the ATP-dependent activator of the B 12 -containing protein CoFeSP reveals how selective protein–protein and protein–cofactor interactions are orchestrated. Furthermore, our results underline the significance of conformational gating during uphill electron transfer and by elucidating the role of the nucleotide, extend our knowledge about biological energy conversions. Obviously, nature has devised different ways of translating the energy stored in the pyrophosphate bond of ATP to enable an energetically unfavourable electron transfer. RACo achieves this task by balancing binding energies with modulations of the coordination sphere of the electron-accepting metal. Materials Chemicals were purchased from Sigma, Fermentas, AppliChem, and Roth and were at least of analytical grade. N 2 and N 2 /H 2 (95%/5%) gases were obtained from Air Liquide. Enzymes (DNA polymerase, DNA ligase and restriction enzymes) were purchased from Thermo Fisher. All anoxic solutions were prepared in bottles with butyl rubber septum by at least four cycles of evacuating and flushing with N 2 gas at a vacuum gas line. Expression and purification Proteins used in this study were prepared as described earlier [4] , [10] , [12] . An optimized purification strategy was employed for CoFeSP used in the ATPase activity to get rid of contaminating ATPases. First, the small subunit (CfsB) was purified in three chromatographic steps from 10 g Escherichia coli BL21(DE3) cells containing the recombinant pPKacsD plasmid as described for CoFeSP [12] . In total, 13 g cells containing pPKacsC were resuspended in 50 mM Tris-HCl, pH 8.0 containing 2 mM dithiothreitol (DTT). After 15-min sonication, the cell lysate was centrifuged for 1.5 h at 35,000 r.p.m. and 10 °C. The supernatant was discarded and the pellet containing the insoluble large subunit CfsA, was successively washed with Tris-buffer containing 1 mM EDTA and centrifuged until the supernatant had become colourless. The washed pellet was resuspended in 10 ml Tris-buffer containing 1 mM DTT. A total of 18 mg of pure CfsB in 2 ml 50 mM Tris-buffer containing 100 μM hydroxocobalamin were mixed with 2 ml of the pellet suspension. The mixture was diluted twofold with Tris-buffer containing 4 M urea and incubated for 15 min at 25 °C. After centrifugation at 12,000 r.p.m. for 10 min, the supernatant was diluted and concentrated to decrease the concentration of urea to less than 0.1 M. Hydroxocobalamin was added to reach a final concentration of 200 μM, and after 45-min incubation at room temperature the mixture was loaded onto a gel filtration column (120 ml Superdex 200 prep-grade, GE Healthcare) equilibrated with 50 mM Tris-HCl, pH 8.0, containing 150 mM of NaCl. Fractions corresponding to the CoFeSP heterodimer were combined, concentrated and frozen in liquid nitrogen. Crystallization For crystallization of the RACo:CoFeSP complex, equimolar amounts of both proteins were incubated in 50 mM Tris-HCl, pH 8.0 containing 150 mM NaCl for 15 min and loaded on a Superdex 200 prep-grade gel filtration column inside a glove box (95% N 2 /5% H 2 ; model B; COY Laboratory Products). Peak fractions corresponding to the size of the RACo:CoFeSP complex from several gel filtration experiments [4] were pooled and concentrated to a final concentration of 35 mg ml −1 . The complex of CoFeSP and its activator RACo was crystallized under anaerobic conditions at 19 °C inside a glove box (95% N 2 /5% H 2 ; model B; COY Laboratory Products). Crystals were grown by sitting-drop vapour diffusion. The protein solution was mixed with same volume of 0.2 M ammonium sulphate, 0.1 M BisTris (pH 6.5) and 25% PEG 3350. After several months, red/brown crystals appeared, which were flash cooled in liquid N 2 with 1,2-butandiol as cryoprotectant. Data collection and structure refinement Diffraction data were collected on BL14.2 operated by the Joint Berlin MX-Laboratory at the BESSY II electron storage ring (Berlin-Adlershof, Germany) at 0.91841 Å wavelength and 100 K temperature [26] . The diffraction data set was integrated and scaled by X-ray detector software [27] . The structure was solved by molecular replacement using Phenix [28] and Phaser [29] with the individual proteins (2YCL [12] , 3ZYY [4] ) as search models. Iterative cycles of model building and refinement were carried out with COOT [30] , Phenix-Refine [28] and CCP4-Refmac [31] . The statistics of data collection and refinement are summarized in Table 1 . Coordinates and structure factors of the reported complex structure have been deposited in the Protein Data Bank (PDB ID 4C1N ). Table 1 Data collection and refinement statistics (molecular replacement). Full size table Isothermal titration calorimetry The interaction of CoFeSP with RACo and Δ100-RACo was investigated by isothermal titration calorimetry using a MicroCal VP-ITC Instrument (MicroCal LLC, Northampton, MA, USA) inside a glove box with N 2 atmosphere and [O 2 ]<0.5 p.p.m. (LabStar, MBraun). All protein samples were prepared in 50 mM Tris-HCl, pH 8.0 containing 150 mM NaCl. A solution of 100 μM RACo or Δ100-RACo was injected into the calorimeter cell containing 10 μM CoFeSP. The spacing time was set to 5 min, stirring speed to 307 r.p.m. Data were analysed with the manufacturers software assuming a ‘one set of sites’-binding model. ATP-dependent activation assay The ATP-dependent reductive activation assay was performed at 25 °C under anoxic conditions (95% N 2 /5% H 2 ; model B; COY Laboratory Products) as described earlier [4] with some modifications: Equimolar concentrations of RACo and CoFeSP were mixed in 100 mM Tris-HCl, pH 7.6 containing 150 mM KCl, 10 mM MgCl 2 and 2 mM DTT. To induce electron transfer from reduced RACo to Co(II)–CoFeSP, 1 mM of Mg-ATP was added. The reduction of CoFeSP was monitored as reported recently [4] . ATPase activity assays A coupled ATPase assay was performed at 25 °C and anoxic conditions (95% N 2 /5% H 2 ; model B; COY Laboratory Products) as described [4] with some modifications. The reaction mixture was prepared in buffer used in the ATP-dependent activation assay (without addition of DTT) containing 2 mM phosphoenolpyruvate, 9.9 units lactate dehydrogenase, 6.8 units PK and 2 μM RACo or CoFeSP, respectively. A complex sample was prepared by mixing equimolar concentrations (2 μM) of RACo and CoFeSP. These solutions served as a blank before 0.16 mM NADH were added to the different samples. Addition of 1 mM ATP initiated the reaction. The rate of ATP hydrolysis was calculated as described [4] . The ATPase activity of RACo in the complex was additionally determined by a modified malachite green-ammonium molybdate assay [32] . The assay solution was prepared by mixing 10 μM of RACo and CoFeSP in 100 mM Tris-HCl, pH 7.6 containing 150 mM KCl, 10 mM MgCl 2 . Reaction was initialized by adding ATP at a final concentration of 5 mM. A sample containing reduced CoFeSP was prepared by incubating CoFeSP with 5 mM DT for 15 min. RACo was added and the reaction was initiated after 10 min by adding ATP. During the time course of 100 min, aliquots were taken and the absorbance of a phosphomolybdate–malachite green complex at 630 nm (Agilent 8453 photodiode array spectrophotometer) was measured. The amount of phosphate released during hydrolysis was calculated from a standard curve prepared by 1−9 nmol of KH 2 PO 4 . As a control, autohydrolysis of ATP in the absence of the proteins was measured and subtracted from the enzyme-catalyzed reaction. The unit of activity was defined as micromoles of Pi released per minute. Redox titration combined with EPR spectroscopy The buffer of protein stock solutions was exchanged to 100 mM CAPSO, pH 9.5 using PD10 columns (GE Healthcare) to extend the negative potential range achievable with sodium dithionite to –600 mV. Samples of a final concentration of 130 μM in 2 ml buffer of RACo, Co(II)–CoFeSP and RACo–Co(II)–CoFeSP complex were prepared. Each sample was repeatedly evacuated and flushed with argon to carefully remove hydrogen gas carried over from protein purification, which might interfere with the Pt electrode measurement. The titration was performed inside a glove box under an atmosphere of nitrogen with traces of remaining oxygen <10 p.p.m. (VAC 101965 OMNI-LAB). A mediator mix containing 50 μM of phenazine methosulphate, toluidine blue, methylene blue, indigocarmine, anthrachinone-2-sulphonate, phenosafranine, safranine T, deiquat, methylviologen and triquat, spanning a range of midpoint potentials from +80 mV to −550 mV, was added to the sample. Sodium dithionite was added stepwise and the potentials were measured with a Schott Pt 5900A platinum redox electrode with internal Ag/AgCl reference. Equilibrium was reached when the measured potential drift was less than 2 mV per minute. For each potential step, exactly 80 μl of the protein solution was quickly transferred into an EPR sample tube, which was then carefully sealed, exported from the glove box and immediately frozen in liquid nitrogen. EPR measurements were performed at 9.3 GHz on a Bruker EMXplus X-band spectrometer equipped with a high sensitivity cylindrical mode resonator (Bruker super-high-Q-cavity, ER 4122 SHQE). Field modulation frequency and amplitude were set to 100 kHz and 10 G, respectively. The temperature was set to 100 K for Co(II) and reduced [2Fe2S] or 10 K for reduced [4Fe4S] using an Oxford ESR 900 helium flow cryostat. Background spectra were recorded for each set of experimental conditions separately on a buffer sample and were subtracted from the protein spectra. Analytical size exclusion chromatography Analytical Size Exclusion Chromatography (Superdex 200 prep-grade gel filtration column) was used to detect the complex formation between Δ60-CoFeSP and RACo. Experiments were performed inside a glove box (95% N 2 /5% H 2 ; model B; COY Laboratory Products). Conditions were described in detail recently [4] . Accession codes: The X-ray crystallographic coordinates for the structure reported in this article have been deposited in the Protein Data Bank (PDB), under deposition numbers 4C1N . These data can be obtained free of charge from the PDB ( http://www.rcsb.org/pdb/home/home.do ). How to cite this article: Hennig, S. E. et al. ATP-induced electron transfer by redox-selective partner recognition. Nat. Commun. 5:4626 doi: 10.1038/ncomms5626 (2014).